Anisotropic breakdown of Fermi liquid quasiparticle excitations in overdoped La2−xSrxCuO4 High-temperature superconductivity emerges from an un-conventional metallic state. This has stimulated strong efforts to understand exactly how Fermi liquids breakdown and evolve into an un-conventional metal. A fundamental question is how Fermi liquid quasiparticle excitations break down in momentum space. Here we show, using angle-resolved photoemission spectroscopy, that the Fermi liquid quasiparticle excitations of the overdoped superconducting cuprate La 1.77 Sr 0.23 CuO 4 is highly anisotropic in momentum space. The quasiparticle scattering and residue behave differently along the Fermi surface and hence the Kadowaki–Wood's relation is not obeyed. This kind of Fermi liquid breakdown may apply to a wide range of strongly correlated metal systems where spin fluctuations are present. Landau theory of Fermi liquids, and its notion of quasiparticles, underlies much of our understanding of how electron interactions affect the properties of a metal [1] . The breakdown of this concept has therefore been studied in great detail by transport and thermodynamic measurements [2] , [3] , [4] , [5] , [6] , [7] , [8] , [9] , [10] . A common assumption is that the Fermi liquid self-energy ImΣ is local, that is, that it depends only on excitation energy ω : and not on momentum ( k ) [11] , [12] . The Fermi liquid breakdown then appears as the cutoff energy ω c vanishes although the electron coupling constant λ and the a priori unknown function F remain constant. There exist relatively few studies of non-local Fermi liquids [13] , [14] , [15] , [16] . CeCoIn 5 is an example of a three-dimensional multi-band material that may have a directional breakdown [17] , [18] . Angle-resolved photoemission spectroscopy (ARPES) is a unique technique to extract the self-energy Σ( k , ω ). It measures an intensity I ( k , ω ) that is proportional to the spectral function A ( k , ω ), a matrix element M ( k , ω ) and the Fermi distribution f ( ω ) [19] . Often matrix elements vary only weakly as a function of ( k , ω ) in which case the ARPES intensity becomes a direct measure of the occupied part of the spectral function, , where ε k is the bare-band dispersion. The self-energy Σ, carrying information about all correlation effects, can be derived experimentally from ImΣ= v k Γ k [20] , [21] , [22] , [23] , where is the bare-band velocity and Γ k is the linewidth of I vs k . Here we demonstrate, using ARPES, that quasiparticle excitations – found in overdoped La 1.77 Sr 0.23 CuO 4 – are strongly anisotropic in momentum space. We find that true Fermi liquid quasiparticles exist around the nodal region, whereas non-Fermi liquid excitations provide a better description of the spectra found near the anti-nodal region (see schematic Fig. 1 ). The quasiparticle scattering and residue are studied as a function of momenta. The simple relation between quasiparticle scattering and mass renormalization proposed by Kadowaki–Wood does not appear to be obeyed. 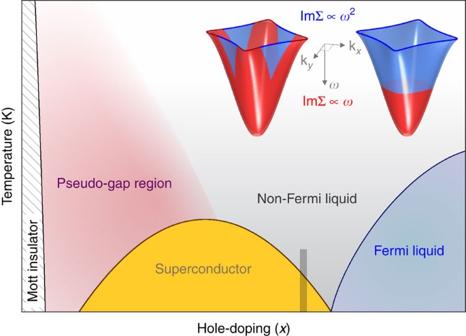Figure 1: Schematic phase diagram of cuprates Doping dependence of the Mott insulating, superconducting, pseudogap and Fermi liquid phase46. A strongly correlated Fermi liquid has a self-energy that scales as Imnear the Fermi surface as illustrated schematically in the top-right inset (blue region). Here we show, using angle-resolved photoemission spectroscopy in the doping regime indicated by the vertical line, that the non-Fermi liquid state appears through an angular breakdown of the Fermi liquid as shown schematically in the top-left inset (blue region). This results in arcs of Fermi liquid quasiparticles separated by gapless non-Fermi liquid excitations (red region in the inset) with. These Fermi liquid arcs are different from the Fermi arcs inside the pseudogap phase as there the arcs are separated by (pseudo) gaped excitations. Notice that around 1/8 doping a Fermi liquid re-entrance is realized47(not shown). Figure 1: Schematic phase diagram of cuprates Doping dependence of the Mott insulating, superconducting, pseudogap and Fermi liquid phase [46] . A strongly correlated Fermi liquid has a self-energy that scales as Im near the Fermi surface as illustrated schematically in the top-right inset (blue region). Here we show, using angle-resolved photoemission spectroscopy in the doping regime indicated by the vertical line, that the non-Fermi liquid state appears through an angular breakdown of the Fermi liquid as shown schematically in the top-left inset (blue region). This results in arcs of Fermi liquid quasiparticles separated by gapless non-Fermi liquid excitations (red region in the inset) with . These Fermi liquid arcs are different from the Fermi arcs inside the pseudogap phase as there the arcs are separated by (pseudo) gaped excitations. Notice that around 1/8 doping a Fermi liquid re-entrance is realized [47] (not shown). Full size image Photoemission spectra ARPES spectra acquired [24] , [25] at T =15 K, from overdoped La 2− x Sr x CuO 4 (LSCO) x =0.23 are shown in Fig. 2a–f . Data were recorded as a series of cuts in momentum space, as indicated in the inset of Fig. 2m . Near the nodal point, the spectra ( Fig. 2a–b ) display a ΔΓ=Γ( ω )−Γ(0) ∝ ω 2 dependence (see Fig. 2g,h ) implying ImΣ ∝ ω 2 as v k varies weakly with ω ( Fig. 2n ). This Fermi liquid property survives up to excitation energies as large as ω ~0.2 eV. For larger ω , a ΔΓ ∝ ω dependence is found (see Fig. 2g,h ). This sudden change from ΔΓ ∝ ω 2 to ∝ ω is accompanied by a marked kink in the dispersion ( Fig. 2n ). 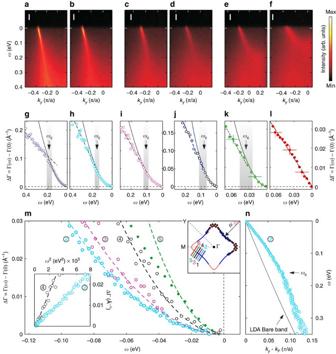Figure 2: ARPES spectra of overdoped La1.77Sr0.23CuO4(LSCO). (a–f) Angle-resolved photoemission intensity as a function of binding energy (ω) and momenta (ky) acquired along the cuts indicated in the top-right inset ofm. The intensities of the spectra were normalized so that they are identical at the momenta indicated by the white bars (seesupplementary Fig. S3). (g–l) Half-width half-maximum linewidth ΔΓ=Γ(ω)−Γ(0) of MDCs vs excitation energy (ω) for spectra shown ina–f. Horizontal and vertical error bars indicate the applied energy resolution and standard deviations, respectively. The vertical grey bands indicate the precision with whichωc– the energy scale below which ΔΓ∝ω2(see alsosupplementary Fig. S4) – can be determined. A zoom on the low-ωpart is shown in panelmwhere the bottom-left inset displays ΔΓ vsω2. The top-right inset ofmindicates the cuts (1–6) and the locus of the gapless excitations with a tight-binding fit (solid line) that is consistent with previous ARPES studies of the Fermi surface in overdoped LSCO48,49. In the present LSCOx=0.23 sample, the areaΥ=1.28 enclosed by the gapless excitations is somewhat larger than the number of carriers48n=1+x=1.23. The doping concentration of the cleaved surface may therefore be slightly larger than that of the bulk. This may explain why no traces of superconductivity was found even though the measurement were carried out atK. (n) Dispersion derived from the MDCs and plotted asvsky−kF. The arrow indicates a kink in the dispersion and the solid line is the bare-band LDA dispersion26witht=0.43 eV. Figure 2: ARPES spectra of overdoped La 1.77 Sr 0.23 CuO 4 (LSCO). ( a – f ) Angle-resolved photoemission intensity as a function of binding energy ( ω ) and momenta ( k y ) acquired along the cuts indicated in the top-right inset of m . The intensities of the spectra were normalized so that they are identical at the momenta indicated by the white bars (see supplementary Fig. S3 ). ( g – l ) Half-width half-maximum linewidth ΔΓ=Γ( ω )−Γ(0) of MDCs vs excitation energy ( ω ) for spectra shown in a – f . Horizontal and vertical error bars indicate the applied energy resolution and standard deviations, respectively. The vertical grey bands indicate the precision with which ω c – the energy scale below which ΔΓ ∝ ω 2 (see also supplementary Fig. S4 ) – can be determined. A zoom on the low- ω part is shown in panel m where the bottom-left inset displays ΔΓ vs ω 2 . The top-right inset of m indicates the cuts (1–6) and the locus of the gapless excitations with a tight-binding fit (solid line) that is consistent with previous ARPES studies of the Fermi surface in overdoped LSCO [48] , [49] . In the present LSCO x =0.23 sample, the area Υ =1.28 enclosed by the gapless excitations is somewhat larger than the number of carriers [48] n =1+ x =1.23. The doping concentration of the cleaved surface may therefore be slightly larger than that of the bulk. This may explain why no traces of superconductivity was found even though the measurement were carried out at K. ( n ) Dispersion derived from the MDCs and plotted as vs k y − k F . The arrow indicates a kink in the dispersion and the solid line is the bare-band LDA dispersion [26] with t =0.43 eV. Full size image Data parametrization Data are parameterized according to the Fermi liquid self-energy (Equation 1) by identifying the Fermi liquid cutoff energy ( ω c ) with the energy scale below which ΔΓ ∝ ω 2 . Furthermore, the bare-band width W =4 t =1.72 eV [26] , obtained from local density approximation (LDA) calculations is used to evaluate bare-band velocity v k . This yields ω c =0.15±0.02 eV and eV −1 for the spectra shown in Fig. 2b . A second result of this parametrization is that F ~ ω provides a better description, of the data, than the commonly made assumption: F =1 (ref. 11 ). Notice that these values of and ω c compare well with those extracted from magneto-resistance measurements on overdoped Tl 2 Ba 2 CuO 6+ x (Tl2201) [27] , [28] . Momentum dependence Continuing the parametrization, using the Fermi liquid self-energy of cuts 1–6 (inset of Fig. 2m ) yields the k -dependence of ω c and . A main result of this work is that both ω c and are strongly anisotropic as a function of momentum k (from hereon expressed by the Fermi surface angle φ , defined in the inset of Fig. 2m ). The energy scale ω c softens rapidly as a function of Fermi surface angle φ and eventually it vanishes at a finite angle φ 0 ≈16° ( Fig. 3a ). At the same time, increases significantly as φ → φ 0 from above (see Fig. 3b ). Thus within the experimental resolution, this marks the complete breakdown of Fermi liquid quasiparticle excitations. This fact is further supported by the observation that ImΣ ∝ ω provides a better description of the data for φ < φ 0 ( Fig. 2l and Supplementary Fig. S1 ). 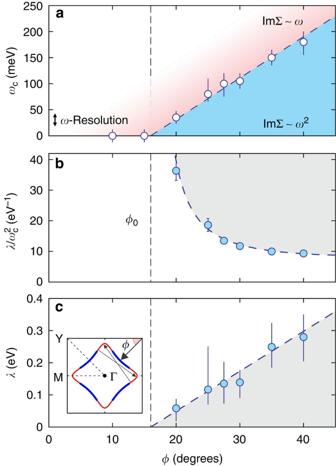Figure 3: Anisotropic Fermi liquid properties (a) Fermi liquid cutoff energyωcderived from momentum distribution analysis (Fig. 2) and plotted vs Fermi surface angleφ. The error bars are the precision with whichωccan be determined from Γkvsω(seesupplementary Fig. S4). The applied energy resolution is indicated in the lower left corner. In the shaded area aboveωc, an approximately linearω-dependence is observed. This region is limited either by the bottom of the valence band or by an interaction cutoff21. (b), whereβ2is obtained from the momentum distribution linewidth ΔΓ=β2ω2andvkis the bare-band Fermi velocity26(see alsosupplementary Table S1and the method section), as a function ofφ. The error bars indicate the standard deviation related to the determination ofβ2. (c) Electron–electron coupling constantλderived fromaandband plotted against Fermi surface angle. The error bars are derived from those shown in panelsaandb. The inset shows schematically the ‘Fermi surface’ consisting of nodal Fermi arcs (blue) where true Fermi liquid quasiparticle excitations are found and the sections with non-Fermi liquid excitations (red). Vertical dashed lines indicateφ0– the Fermi surface angle whereωc→0. All other dashed lines are guides to the eye. Figure 3: Anisotropic Fermi liquid properties ( a ) Fermi liquid cutoff energy ω c derived from momentum distribution analysis ( Fig. 2 ) and plotted vs Fermi surface angle φ . The error bars are the precision with which ω c can be determined from Γ k vs ω (see supplementary Fig. S4 ). The applied energy resolution is indicated in the lower left corner. In the shaded area above ω c , an approximately linear ω -dependence is observed. This region is limited either by the bottom of the valence band or by an interaction cutoff [21] . ( b ) , where β 2 is obtained from the momentum distribution linewidth ΔΓ= β 2 ω 2 and v k is the bare-band Fermi velocity [26] (see also supplementary Table S1 and the method section), as a function of φ . The error bars indicate the standard deviation related to the determination of β 2 . ( c ) Electron–electron coupling constant λ derived from a and b and plotted against Fermi surface angle. The error bars are derived from those shown in panels a and b . The inset shows schematically the ‘Fermi surface’ consisting of nodal Fermi arcs (blue) where true Fermi liquid quasiparticle excitations are found and the sections with non-Fermi liquid excitations (red). Vertical dashed lines indicate φ 0 – the Fermi surface angle where ω c →0. All other dashed lines are guides to the eye. Full size image Not only does the self-energy change from ω 2 to ω , the scattering is generally increasing upon moving from the nodal towards the anti-nodal region. This is consistent with angle-dependent magneto-resistance experiments on overdoped Tl2201 [4] . ARPES experiments on overdoped Tl2201 have, however, reported the opposite trend [29] . The origin of this discrepancy remains an open question. The angular breakdown of Fermi liquid quasiparticles implies that the Fermi surface consists of (FL) Fermi arcs connected by gapless non-Fermi liquid quasiparticle excitations ( Fig. 3c inset). Notice that these Fermi arcs are different from the Fermi arcs found inside the pseudogap phase of underdoped cuprates [30] . In fact, the last mentioned arcs are typically not composed of Fermi liquid quasiparticles [31] in the strict sense imposed here and the arcs are separated by gaped excitations [32] . It is, however, not impossible that there is a connection between the non-Fermi liquid like excitations and the pseudogap. The ‘broken’ Fermi surface could, for example, be a precursor to the pseudogap phase. The momentum dependence of ω c and implies that also λ has a strong dependence on the Fermi surface angle (see Fig. 3c ). This strongly suggest that λ and ω c are coupled parameters. Within error bars, λ ∝ ω c as predicted for two-dimensional Fermi liquids in the presence of spin fluctuations [33] , [34] . In this context, it is interesting to notice that the broken Fermi surface sections are connected by the incommensurate antiferromagnetic spin excitation wavevectors [35] observed by neutron spectroscopy [36] (see inset Fig. 3c ). It is, however, not impossible that disorder [37] also contributes to the Fermi liquid breakdown. The elastic scattering, presumably originating from impurities, increases dramatically across the Fermi liquid breakdown as shown in Supplementary Fig. S2 . Nonetheless, spin fluctuations appear as the most plausible driving mechanism for the anisotropic Fermi liquid breakdown. Kramers–Kronig transforming ImΣ yields the real part of the self-energy ReΣ and hence the quasiparticle residue Z ≡ (1−∂ReΣ/∂ ω ) −1 . In the most simple case where λ and F =1 are constants, Z ∝ ω c is found [11] , [13] . This leads to the Kadowaki–Woods relation [11] , [13] ( ) between the quasiparticle residue Z and the electron scattering amplitude . However, in our case neither λ nor F is a constant. A Kramers–Kronig transformation of a self-energy, that has ω c ∝ λ and F ∝ ω , yields . Consequently, the Kadowaki–Woods relation cannot be obeyed. We also notice that is consistent with theories of itinerant electrons near a magnetic quantum critical point [14] , [38] . In this scenario, ω c is a measure of the distance to the so-called hot spot [38] , [39] . This kind of quantum criticality predicts a logarithmic divergent thermopower , where T is the temperature [38] . Such a temperature dependence has been reported [40] , [41] for La 2− x − y R y Sr x CuO 4 with R=Eu ( y =0.2) or Nd ( y =0.4) and dopants x =0.24 comparable to this study. As pointed out in recent numerical studies, the vicinity of the van-Hove singularity to the Fermi level should not be neglected and in concert with electron correlation this can also produce non-Fermi liquid behaviour [42] , [43] . LSCO sample The LSCO with x =0.23 ( T c =25 K) sample used for this ARPES study was grown by the floating zone method at Bristol University. The quality of the current LSCO x =0.23 single crystal has been demonstrated in previous publications. Resistivity curves in high magnetic field showed a residual resistivity of ρ 0 ≈20 μΩ cm (ref. 2 ). The spin excitation spectrum was probed by inelastic neutron spectroscopy [44] and the excellent superconducting properties of these samples were demonstrated by a small angle neutron scattering study of the vortex lattice [45] . ARPES experiments The ARPES experiments were carried out at the Swiss Light Source on the surface and interface spectroscopy beam line [24] using 55 eV circular polarized photons. The sample was cleaved at T =15 K by employing a cleaving tool [25] operated in situ in the sample space kept under ultra high vacuum (10 −11 mbar). The photoemitted electrons were analysed by a SCIENTA 2002 electron analyser configured to have a 0.15° angular resolution as in Chang et al . [21] Different detector channel efficiencies were normalized by measuring a spectrum on poly-crystalline copper in thermal and electrical contact with the sample. The Cu-spectra were also used to extract (i) the chemical potential μ and (ii) the overall energy resolution Δ E ≈24 meV for the experimental setup. All ARPES spectra reported in this work were recorded in the second Brillouin zone but are, for convenience and clarity of display, presented by their equivalent cuts in the first zone. Elastic scattering The elastic momentum distribution curve (MDC) linewidth Γ 0 ( φ ) sharpens rapidly as the Fermi surface angle φ is varied towards the nodal direction ( φ → π /4), see Supplementary Fig. S2 . This is consistent with previous reports on LSCO, for this and other dopings [49] . Note that the linewidth Γ 0 ( φ ≈ π /4)=0.028 Å −1 reported here, is somewhat sharper than what we reported for underdoped LSCO x =0.145, and also sharper than Γ 0 ( φ ≈ π /4)≈0.05 Å −1 reported in Yoshida et al . [49] . The elastic MDC linewidth Γ 0 originates, most likely, from scattering due to impurities [50] . The sharpness of Γ 0 can therefore be taken as evidence for high sample quality. The measured elastic linewidth can be modelled as , where Å −1 is the instrumental momentum resolution and Γ i (0) is the intrinsic elastic scattering. We find that Γ 0 ≈2Γ r near the nodal point and hence . The elastic MDC linewidth is therefore fully resolved with the applied momentum resolution of 0.15°, see Supplementary Fig. S2 . Elastic and inelastic scattering usually originates from fundamentally different processes. To first approximation, the self-energy therefore becomes a sum of the two: ImΣ=ImΣ elastic +ImΣ inelastic [11] , [12] , [27] . The elastic component is commonly assumed to be independent of energy ( ω ) and temperature T , but may depend on momentum (see Supplementary Fig. S2 ). These assumptions were applied, throughout this paper, to disentangle elastic and inelastic contributions. In Supplementary Fig. S1 , it is shown how an alternative modelling ( ) provides a poor description of the observed data. Electronic band structure The band structure of La 1.77 Sr 0.23 CuO 4 can be parameterized by a tight binding model: where μ is the chemical potential, and t , t 1 and t 2 denote nearest, second-nearest and third-nearest neighbour hopping integrals on a square lattice, respectively. The ratios μ / t =0.86, t 1 / t =−0.136, t 2 / t =0.068, t 3 / t =0 and t 4 / t =−0.02 are chosen such that fits the marginal Fermi surface as shown in Fig. 2m . The bare band is herein modelled by using the LDA bandwidth W =4 t =1720, meV (ref. 26 ). How to cite this article: Chang, J. et al . Anisotropic breakdown of Fermi liquid quasiparticle excitations in overdoped La 2− x Sr x CuO 4 . Nat. Commun. 4:2559 doi: 10.1038/ncomms3559 (2013).